Manipulating microRNAmiR408enhances both biomass yield and saccharification efficiency in poplar The conversion of lignocellulosic feedstocks to fermentable sugar for biofuel production is inefficient, and most strategies to enhance efficiency directly target lignin biosynthesis, with associated negative growth impacts. Here we demonstrate, for both laboratory- and field-grown plants, that expression of Pag-miR408 in poplar ( Populus alba × P. glandulosa ) significantly enhances saccharification, with no requirement for acid-pretreatment, while promoting plant growth. The overexpression plants show increased accessibility of cell walls to cellulase and scaffoldin cellulose-binding modules. Conversely, Pag-miR408 loss-of-function poplar shows decreased cell wall accessibility. Overexpression of Pag-miR408 targets three Pag-LACCASES , delays lignification, and modestly reduces lignin content, S/G ratio and degree of lignin polymerization. Meanwhile, the LACCASE loss of function mutants exhibit significantly increased growth and cell wall accessibility in xylem. Our study shows how Pag-miR408 regulates lignification and secondary growth, and suggest an effective approach towards enhancing biomass yield and saccharification efficiency in a major bioenergy crop. Plant cells walls are the primary source of terrestrial biomass and lignocellulosic biomass has been considered an important source of simple sugars for downstream conversion. Crop traits can be optimized by regulating single genes to achieve significantly increased yield or stress resistance [1] , [2] , [3] , [4] , [5] . Moreover, engineering plants cell walls for more efficient deconstruction is becoming a central technology in the generation of biofuels and bio-based chemicals and materials from lignocellulosic biomass [6] , [7] , [8] , [9] . The approach usually targets structural genes involved in the biosynthesis of cell wall polymers, the most common target being the lignin polymer [10] , [11] . However, genetically engineered low-lignin plants are often weak, stunted and produce less total biomass [12] , [13] , [14] . This may be due to lack of lignin deposition in critical cells such as xylem, tracheary elements, and vessels [15] , altered biosynthesis of related secondary metabolites (flavonoids, coumarins, and lignans) that might influence plant growth and development [13] , [16] , or ectopic activation of defense responses with associated growth trade-offs [14] , [17] . Approaches to overcoming the growth defects in lignin-modified plants have included screening for suppressor mutations [13] , blocking defense signaling pathways [17] , restoring lignification to critical vascular tissues [15] , [18] , and generating haplo-insufficient alleles through gene editing [15] . In these cases, the resulting plants still exhibit small yield penalties. Techno-economic analysis reveals that yield, rather than cell wall compositional parameters, is the critical factor in the economic viability of a bioenergy crop such as poplar ( Populus spp) [19] . There is therefore a need to develop strategies for biomass engineering that can combine reduced cell wall recalcitrance with enhanced yield. One approach is to harness genetic changes that pleiotropically affect secondary growth parameters. MicroRNAs (miRNA), endogenous small noncoding RNAs of 21–24 nucleotides in length, are key eukaryotic gene regulators that play critical roles in plant development and stress tolerance [20] , and some have targets that may be involved in secondary wall formation and lignification [21] , [22] . miR408 is a highly conserved miRNA of 21 nucleotides, first identified in Arabidopsis thaliana [23] . Its over-expression increases biomass and seed yield in Arabidopsis and rice, potentially through effects on the copper-containing proteins plantacyanin and laccase [24] . These growth effects, coupled with the suggestion of laccase as a target, suggest the possibility that manipulating miR408 might overcome the growth defects caused by the down-regulation of lignin synthesis through direct targeting of structural genes. Here, we show that overexpression of Pag-miR408 in hybrid poplar targets three LACCASES , co-down-regulation of which can significantly improve plant growth but also increase cell wall saccharification efficiency without acid pretreatment, as confirmed by using genome editing to simultaneously knock out all three targets of Pag-miR408 . Although the associated changes in lignin properties as a result of Pag-miR408 overexpression are only modest, the large increase in saccharification efficiency is associated with changes in xylem development that may lead to increased accessibility of cell walls to hydrolytic enzymes. This work demonstrates the potential of manipulating non-coding RNA to achieve both enhanced biomass and reduced cell wall recalcitrance, critical for the development of an environmentally friendly lignocellulosic biofuels industry. Overexpression of miR408 enhances biomass yield We generated overexpression ( miR408_OX ) and miR408 -knockout poplars using a CRISPR/Cas9 genome editing approach (Supplementary Fig. 1a, b ). After statistical analysis of plant height and stem diameter in three independent miR408_OX lines (#1, #5, and #6) (Supplementary Fig. 1c ), two independent homozygous lines which had 218 bp genomic deletions ( miR408_cr #8 and #20) were selected for further study (the identification of miR408 _ cr poplar is shown in Supplementary Fig. 2 ). The miR408_OX poplars displayed similar phenotypes of significantly increased plant height (34.75%, 20.42%, 16.94%) (Fig. 1a, b ) and stem diameter (27.80%, 15.83%, 11.38%) (Fig. 1c ), whereas the knockout lines showed no obvious changes in these parameters (Fig. 1a-c ). In addition, overexpression or knockout of miR408 did not result in a change of internode number compared with WT (Supplementary Fig. 1d ). The net photosynthetic rate (NPR) of miR408_OX lines was nearly 40% higher than that of WT, whereas no significant difference between WT and knock-out lines was observed (Supplementary Fig. 1e ). Fig. 1: Overexpression of miR408 enhances biomass yield, cell wall accessibility and saccharification efficiency in poplar. a Growth phenotypes of miR408 overexpression and knockout lines. Bar, 15 cm. b , c Comparisons of plant height and basal stem diameter for the above lines. The upper and lower whiskers represent the maximum and minimum values, respectively. The upper, lower and middle box lines represent the two quartiles and median of values in each group. All P -values are from two-tailed Student’s t -tests, n represents 11 to 21 trees sampled respectively from WT ( n = 21), miR408_OX #1 ( n = 13), #5 ( n = 11), #6 ( n = 11), miR408_cr #8 ( n = 11), #18 ( n = 11) and #20 ( n = 11). d Comparison of vascular cambium zones and xylem area. Scale bar, 50 μm (upper); 100 μm (down). xy, xylem; ca, cambium; ph, phloem. Ten samples each were analyzed with similar results. e Fluorescence microscopy of cell walls exposed to Tr CBM1-GFP from WT, miR408_OX #1, miR408_cr #20 and CCR2 -RNAi tissue cultured lines. The CCR2 -RNAi line was used as the positive control. Tr CBM1 specifically recognizes cellulose and the probe exhibits green fluorescence. Autofluorescence (red) under UV shows lignin and the merged images highlight the negative correlation between probe binding and autofluorescence. Scale bars, 100 μm. f Fluorescence microscopy of transverse sections of one-year-old natural dried poplar stems from WT and miR408_OX exposed to dye-bound cellulases for 24 h. The overexpression lines showed much stronger green fluorescence than WT. Scale bars, 100 μm. Xy, xylem; pi, pith. g , h Histograms showing relative green fluorescence intensity of Tr CBM1-GFP ( g ) and dye-bound cellulase ( h ). i Saccharification efficiency of WT and miR408_OX plants without pretreatment. Values are presented as means ± SD ( n = 3, All P -values are from two-tailed Student’s t -tests; n represents 3 transgenic lines, and three replicate samples were carried out for each transgenic line). Source data are provided as a Source Data file. Full size image qRT-PCR analysis revealed that mature miR408 transcript was mainly present in mature leaves, young stems and roots (Supplementary Fig. 3a ). In vascular tissue, miR408 transcripts were highly expressed in vascular cambium and developing xylem, with the lowest expression in mature xylem (Supplementary Fig. 3a ). To provide further insights into miR408 expression pattern in the above organs, a 2-kb promoter region of miR408 was fused with GUS gene and transformed into poplar. GUS signal was detected in leaf veins (Supplementary Fig. 3b, c ) and in root vascular tissue (Supplementary Fig. 3d ). Promoter activity of miR408 was mainly detected in the vascular cambium that will differentiate into xylem, but was weak in mature xylem (Supplementary Fig. 3e-g ). Semi-thin sectioning showed that cells in the secondary xylem of miR408_OX plants were enlarged (Fig. 1d ). The cambium zone of miR408_OX lines was wider by about 42% (Fig. 1d , Supplementary Fig. 4a ). Compared with WT, miR408_OX showed more xylem cells, xylem area (Supplementary Fig. 4b, c ) and vessels (Supplementary Fig. 4d, e ). Statistical analysis showed that vessel cell area in miR408_OX was significantly greater than in WT (Supplementary Fig. 4f, g ), whereas there were no differences in fiber cell area (Supplementary Fig. 4h ). Overexpression of miR408 enhances saccharification efficiency To test whether the enlarged xylem cells might possess more loosely-organized cell walls, we utilized green fluorescent protein (GFP)-tagged CBM1/3 ( Ct CBM3-GFP and Tr CBM1-GFP) to identify exposed cellulose surfaces. The carbohydrate-binding module Ct CBM3 derived from the Cladosporium thermocellum cellulosomal scaffoldin protein (CipA) and Tr CBM1 derived from T . reesei cellobiohydrolase I specifically recognize the planar face of crystalline cellulose [25] , [26] . The area and intensity of the green fluorescence signal from Tr CBM1-GFP binding was much greater in tissue-cultured miR408_OX poplar than in the WT (Fig. 1e ). Moreover, the green fluorescence signal appeared to cover a larger area of xylem tissues than in the CCR2 -RNAi positive control (Fig. 1e, g ), which has significantly enhanced saccharification [27] . However, the miR408 knockout line #20 showed a very weak green fluorescence signal (Fig. 1e, g ). Similarly increased cell wall accessibility of cellulose microfibrils to cellulase enzymes was seen for Tr CBM1-GFP (Supplementary Fig. 5a ) and Ct CBM3-GFP (Supplementary Fig. 5b ) binding to one-year-old natural dried poplar stems grown in the greenhouse. Notably, the labeling was highest in areas with reduced lignin (red autofluoresence) content. Next, we examined the ability of green dye-labeled cellulase enzyme to bind to poplar stem cross sections. Unlike the CBM1/3-GFP labeling, all of the cell walls were labeled irrespective of the presence of lignin. However, the green fluorescence was very weak in the WT and much stronger in the miR408_OX plants, indicating strongly increased accessibility of cellulase to the cell walls of miR408_OX plants (Fig. 1f, h ). Furthermore, in the cross sections of natural dried one-year-old poplar stems, the miR408_OX plants showed many more collapsed cells, probably due to water loss (Supplementary Fig. 6 ), whereas the cells were not collapsed in the cross sections of fresh material of the same lines (Supplementary Fig. 7 ). Saccharification efficiency was determined by measuring the release of sugars from cell walls directly by digestion with cellulase, without acid pretreatment. The one-year-old natural dried poplar cell walls of the miR408_OX lines contained a slightly higher percentage of total sugars than the controls (Supplementary Fig. 8a ). The total amount of enzyme-released sugar increased by 110-115% in the three miR408_OX lines (Supplementary Fig. 8b ). When calculated as a percentage of total cell wall sugar, saccharification efficiency increased by 85-92% in the miR408_OX lines compared with the WT (Fig. 1i ). Overexpression of miR408 enhances biomass yield and accessibility to Tr CBM1-GFP of field-grown plants After one-year growth in the field, the miR408_OX poplars displayed similar phenotypes of significantly increased plant height (42.57%, 41.06%, 38.20%) (Fig. 2a, b ) and stem diameter (35.70%, 33.29%, 31.30%) (Fig. 2c ) as seen with the greenhouse-grown poplars. Tr CBM1-GFP binding results showed the area and intensity of the green fluorescence signal was much stronger in the miR408_OX poplars (Fig. 2d ), indicating the significantly increased cell wall accessibility of cellulose microfibrils to cellulase enzymes. Fig. 2: Overexpression of miR408 enhances biomass yield, cell wall accessibility and saccharification efficiency in field-grown plants. a Growth phenotypes of miR408 overexpression lines in the field. Bar, 90 cm. b , c Comparisons of plant height and basal stem diameter for the above lines. The upper and lower whiskers represent the maximum and minimum values, respectively. The upper, lower and middle box lines represent the two quartiles and median of values in each group. All P -values are from two-tailed Student’s t -tests. n represents 10-21 trees sampled respectively from WT ( n = 21) and miR408_OX #1, #5, #6 ( n = 10). d Fluorescence microscopy of cell walls exposed to Tr CBM1-GFP from WT and miR408_OX poplars grown in the field. Bar, 100 μm. Six samples each were analyzed with similar results. Source data are provided as a Source Data file. Full size image miR408 alters lignin deposition in poplar Cross-sections with phloroglucinol staining showed that the basal stem xylem width of miR408_OX plants was significantly increased compared to WT (Fig. 3a , Supplementary Fig. 9a ). No significant difference in secondary cell wall thickness of vessels and fibers was observed between miR408_OX and WT plants, but thickness was decreased by around 50% in knockout poplars (Fig. 3b , Supplementary Fig. 9b ). RNA-seq data showed that the expression levels of cell wall related NAC TFs such as VND7 and SND1 were down-regulated in miR408_cr poplar, and a negative cell wall related TF LBD15 was highly up-regulated in miR408_cr poplar (Supplementary Fig. 9c ). To determine whether the above changes in vascular morphology and saccharification efficiency were associated with changes in lignin deposition, we analyzed cross-sections from the first (IN1) to the eighth internode (IN8) with phloroglucinol staining (Supplementary Fig. 9d ). Statistical analysis (Supplementary Fig. 9d, e ) confirmed significantly reduced number of lignified xylem cells, indicative of delayed secondary xylem differentiation, in miR408_OX compared with WT, with slightly increased number of xylem cells in knock-out poplars. Fig. 3: miR408 overexpression alters lignin deposition in poplar. a Cross-sections of six-month-old basal stems of WT, overexpression and knockout poplar lines. Stem cross-sections were stained with phloroglucinol-HCl (red color indicates lignin). Scale bar, 1 mm. Ten samples each were analyzed with similar results. b Cell wall ultrastructure of mature xylem. Scale bar, 5 μm. Six samples each were analyzed with similar results. c CRM images of lignin in IN20 secondary xylem cell walls. The scale bar from 200 – 800 represents signal intensity from low to high. The red color represents a higher signal intensity than blue. Lignin is deposited throughout the cell wall in WT, whereas it is localized more in the corners of the cell walls of miR408_OX plants, indicating that miR408_OX plants have delayed lignification. Six samples each were analyzed with similar results. d-g 2D-HQSC NMR spectra revealing aromatic regions ( d, f ) and lignin aliphatic side chain regions ( e, g ). The lignin in miR408_OX poplar lines had a lower relative abundance of S lignin units and a correspondingly higher abundance of G lignin units. The β-aryl ether subunits (A) were lower in miR408_OX poplars. Full size image To understand the relationship between altered cell wall morphology and the changes in bulk lignin levels, we employed confocal Raman microspectroscopy (CRM) and stimulated Raman scattering (SRS). CRM and SRS techniques are applied to reveal the spatial distribution of intact plant cell wall components in their native form [28] . Stem cross-sections were analyzed using internode 20 (IN20), integrating over the 1600 cm −1 band (1550 –1 to 1640 cm −1 ) dominated by the aromatic C-C vibration (Fig. 3c ). The lignin signal intensity in the secondary xylem cell walls in IN20 of miR408_OX plants was weak compared with that of WT plants (Fig. 3c ), indicating a reduced lignin content. Furthermore, SRS with the quantitative analysis presented as pixel intensity showed that the SRS intensity of lignin across the cell wall was weaker in IN5-20 of m iR408 plants than in the corresponding internodes of WT plants (Supplementary Fig. 10 ). Two-dimensional heteronuclear single quantum coherence nuclear magnetic resonance (2D-HSQC NMR) spectroscopy was performed on isolated lignin, using double enzymatic digestion. Only trace levels of H lignin units were detected. Lignin in miR408_OX lines had a lower relative abundance of S lignin units and a correspondingly higher abundance of G lignin units (Fig. 3d, f ). The S/G ratio in three independent miR408_OX plants was 1.98, 2.02 and 2.21, compared with 2.88 in WT poplar (Fig. 3d ). β-Aryl ether subunits (A) in miR408_OX poplars were relatively lower than in WT (Fig. 3e, g ). 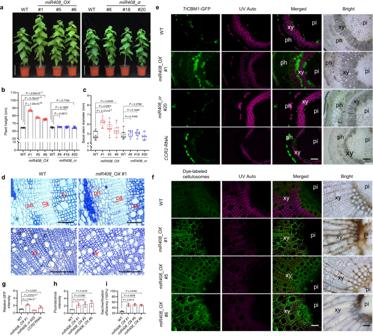Fig. 1: Overexpression ofmiR408enhances biomass yield, cell wall accessibility and saccharification efficiency in poplar. aGrowth phenotypes ofmiR408overexpression and knockout lines. Bar, 15 cm.b,cComparisons of plant height and basal stem diameter for the above lines. The upper and lower whiskers represent the maximum and minimum values, respectively. The upper, lower and middle box lines represent the two quartiles and median of values in each group. AllP-values are from two-tailed Student’st-tests, n represents 11 to 21 trees sampled respectively from WT (n= 21), miR408_OX #1 (n= 13), #5 (n= 11), #6 (n= 11), miR408_cr #8 (n= 11), #18 (n= 11) and #20 (n= 11).dComparison of vascular cambium zones and xylem area. Scale bar, 50 μm (upper); 100 μm (down). xy, xylem; ca, cambium; ph, phloem. Ten samples each were analyzed with similar results.eFluorescence microscopy of cell walls exposed toTrCBM1-GFP from WT,miR408_OX#1,miR408_cr#20 andCCR2-RNAi tissue cultured lines. TheCCR2-RNAi line was used as the positive control.TrCBM1 specifically recognizes cellulose and the probe exhibits green fluorescence. Autofluorescence (red) under UV shows lignin and the merged images highlight the negative correlation between probe binding and autofluorescence. Scale bars, 100 μm.fFluorescence microscopy of transverse sections of one-year-old natural dried poplar stems from WT andmiR408_OXexposed to dye-bound cellulases for 24 h. The overexpression lines showed much stronger green fluorescence than WT. Scale bars, 100 μm. Xy, xylem; pi, pith.g,hHistograms showing relative green fluorescence intensity ofTrCBM1-GFP (g) and dye-bound cellulase (h).iSaccharification efficiency of WT andmiR408_OXplants without pretreatment. Values are presented as means ± SD (n= 3, AllP-values are from two-tailed Student’st-tests; n represents 3 transgenic lines, and three replicate samples were carried out for each transgenic line). Source data are provided as a Source Data file. Furthermore, the distribution of β–β (B) regions differed significantly between miR408_OX and WT plants (Supplementary Table 1 ). Because β- O −4 linkages are strongly correlated with S lignin, and a lower level of β- O −4 corresponds to a lower S/G ratio [29] , these data are consistent with the compositional data revealed by correlations in the aromatic region. To further quantify lignin and other cell wall polymers in miR408_OX poplars, woody stem tissues were analyzed using a range of wet chemistry approaches. Overall, the miR408_OX poplars showed a 10% decrease in lignin content compared with WT using the acetyl bromide (AcBr) method (Supplementary Fig. 11 ). The results obtained from Klason method revealed that the contents of both acid-insoluble lignin (AIL) and acid-soluble lignin (ASL) were decreased in miR408_OX stem compared with that in WT, with a decrease in total Klason lignin of around 4% (Table 1 ). Analysis of total cell wall carbohydrates indicated little change in cell wall glucose levels (reflecting cellulose), but reductions in xylose, mannose and glucuronic acid (reflecting hemicelluloses) in miR408_OX stem compared with that in WT (Table 1 ). 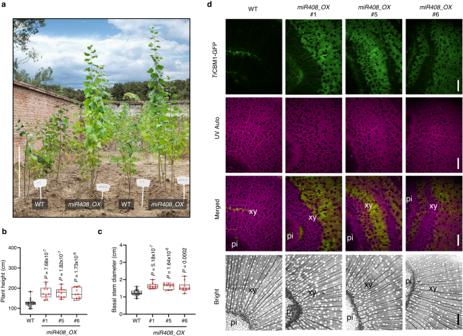Fig. 2: Overexpression ofmiR408enhances biomass yield, cell wall accessibility and saccharification efficiency in field-grown plants. aGrowth phenotypes ofmiR408overexpression lines in the field. Bar, 90 cm.b,cComparisons of plant height and basal stem diameter for the above lines. The upper and lower whiskers represent the maximum and minimum values, respectively. The upper, lower and middle box lines represent the two quartiles and median of values in each group. AllP-values are from two-tailed Student’st-tests. n represents 10-21 trees sampled respectively from WT (n= 21) andmiR408_OX#1, #5, #6 (n= 10).dFluorescence microscopy of cell walls exposed toTrCBM1-GFP from WT andmiR408_OXpoplars grown in the field. Bar, 100 μm. Six samples each were analyzed with similar results. Source data are provided as a Source Data file. Table 1 Cell wall composition of WT and miR408_OX poplars Full size table Analysis of acetylated lignin samples by gel permeation chromatography (GPC) method revealed reductions in the weight-average (Mw) and number-average (Mn) molecular weights, with increased poly-dispersity indexes (Mw/Mn), in miR408_OX compared to WT poplars (Table 2 ). Table 2 Weight-average molecular weight (Mw), number-average molecular weight (Mn), and poly-dispersity indices (PDI, Mw/Mn) of acetylated lignin samples from WT and miR408_OX poplars Full size table miR408 targets LAC19, LAC25 and LAC32 To investigate the target(s) of miR408 that influence cell wall structure and composition, RNA-seq analysis was performed on stems of overexpression lines (#1 and #6), CRISPR-Cas9 knock-out lines ( miR408_cr #8 and #20) and WT poplars. We identified a total of 12,166 differentially expressed genes (DEGs) (Fig. 4a , Supplementary Fig. 12a ). The down-regulated DEGs in miR408_OX poplars were enriched to the phenylpropanoid biosynthesis pathway (Fig. 4b , Supplementary Fig. 12b, c ), indicating miR408 may be involved in lignin biosynthesis. In the miR408_cr poplar, the expression of key genes in lignin biosynthesis such as COMT1 and CCoAOMT were nearly 2.3 times higher than that of WT plants, and the phenylpropanoid pathway genes, including PAL1/2 and C4H were also up-regulated with fold change values 2.5 and 2.8, respectively (Supplementary Fig. 12c ). These results indicated that lignin biosynthesis pathway is more active in miR408_cr plants, which is consistent with the increased intensity of phloroglucinol staining (Supplementary Fig. 9d ). Using psRNAtarget prediction, three LACCASES , LAC19 , LAC25 , LAC32 were predicted as the highest potential targets of miR408 (Fig. 4c , Supplementary Data 1 ). qRT-PCR results showed LAC19 , LAC25 and LAC32 transcripts were significantly decreased in miR408_OX plants while not obviously changed in miR408_cr poplars (Fig. 4d ). This may be because the five predicated LACs, namely LAC19 , LAC25 , LAC32 , LAC47 and LAC55 were also predicted to be targeted by at least one of the microRNAs such as miR475 , miR396 , miR1447 , miR397 , miR169 , miR7826 , miR7466 and miR7817 (Fig. 4c ). There was no significant change in the transcript level of LAC47 and LAC55 in RNA-seq data (Supplementary Fig. 12d ) or as determined by qRT-pCR (Supplementary Fig. 12e ). Phylogenetic analysis indicated that Potri.013G152700 ( PtrLAC32 ) is a homolog of LAC13 of A. thaliana , a target of miR408 [30] . Potri.008G073800 ( PtrLAC19 ) and Potri.010G183500 ( PtrLAC25 ) share the highest homology and are closely related to LAC12 in A. thaliana (Supplementary Fig. 13 ). Fig. 4: miR408 targets LAC19, LAC25 and LAC32 . a Venn diagram comparison from RNA-Seq data analysis of miR408_OX and miR408_cr poplars. b KEGG pathway enrichment of DEGs that are down-regulated in miR408_OX poplars. c An interaction network of five predicated LACs ( LAC19 , LAC25 , LAC32 , LAC47 and LAC55 ) with miR408 and other miRNAs. The thickness of the green line represents the strength of the interaction. d qRT-PCR showing the relative transcript levels of LAC19 , LAC25 and LAC32 with high score using psRNAtarget in WT and miR408_OX and knockout plants. Values are means ± SD (All P -values are from two-tailed Student’s t -tests., n represents 3 trees sampled respectively from miR408_OX #1, miR408_OX #6, miR408_cr #8 and miR408_cr #20). e–g 5’RACE assays showed the cleavage site of the LAC19 ( e ), LAC25 ( f ) and LAC32 ( g ). The red lines in exon 2 show the target sites, and the black arrows show the detailed miR408-guided cleavage positions. h , i Localization of LACs and Pag-miR408 using FISH method. Specific probes were designed to label miR408 , LAC19 and LAC25 as green, pink and red, respectively. Lignin autofluorescence is displayed in blue. The merged images showed spatial correspondence between miR408 and LAC19 and LAC25 . In young stem ( h ), miR408 was expressed in all the tissues, while LAC25 was highly expressed in xylem and epidermal cells, and slightly expressed in phloem cells; LAC19 was only expressed in the epidermis and parenchyma cells. In mature stem ( i ), miR408 was expressed in all the tissues, while LAC25 was highly expressed in xylem, phloem fiber and cortical cells; LAC19 was expressed in cortical and parenchyma cells, but not in phloem fiber or xylem cells. Scale bar, 20 μm. Three samples each were analyzed with similar results. The dashed box represents phloem fibers. Arrows indicate the epidermis. Boxes in h and i represent the enlarged area of cambium and cortex, respectively. Source data are provided as a Source Data file. Full size image Extractable laccase protein levels of miR408_OX plants were approximately 22.5 % lower on average than in WT (Supplementary Fig. 12f ). LAC19, LAC25 and LAC32 were highly expressed in stems and root (Supplementary Fig. 12g-i ), which are highly lignified tissues. In vitro assays using effector-reporter system of luciferase (Supplementary Fig. 14a, b ) confirmed that miR408 can negatively regulate the expression of LAC19, LAC25 and LAC32 . Based on 5´ RACE assay of LAC19 (Fig. 4e ), the issue 7/20 means that seven of twenty clones from the PCR products contained an miR408 -guided cleavage 5´ end that mapped precisely to exon 2. Based on 5´ RACE assays of LAC25 (Fig. 4f ) and LAC32 (Fig. 4g ), the cleavage sites were all located at exon 2, and six and seven, respectively from the twenty PCR products mapped precisely to the cleavage sites. To verify the possibility of spatial interactions between miR408 and LACs , fluorescence in situ hybridization (FISH) was carried out. Specific probes (FAM, CY5 and CY3) were designed to label miR408 , LAC19 and LAC25 as green, pink and red, respectively. Lignin autofluorescence showed as the blue signal. In young stems, miR408 was expressed in all the tissues, whereas LAC25 was highly expressed in xylem and epidermal cells, and weakly expressed in phloem cells; LAC19 was only expressed in the epidermal and parenchyma cells (Fig. 4h ). In mature stems, miR408 was expressed in all tissues, whereas LAC25 was highly expressed in xylem, phloem fiber and cortical cells. LAC19 was expressed in cortical and parenchyma cells, not in phloem fiber or xylem cells (Fig. 4i ). The merged images of miR408 and LACs showed there is a spatial correlation between miR408 and LAC19 and LAC25 , and merged images of lignin and LACs are consistent with the involvement of the LACs in lignification. lac19 lac25 lac32 poplar shows enhanced growth and saccharification efficiency To explain the improvement of saccharification efficiency in miR408 _ OX poplar at the molecular level, we designed four sgRNAs to target LAC19 , LAC25 and LAC32 (Supplementary Fig. 15a ) to generate lac19 lac25 lac32 loss-of-function plants. Meanwhile, we also constructed a LAC19 , LAC25 and LAC32 vector to generate LACs overexpression poplar (Supplementary Fig. 15b ). After PCR and sequencing, we obtained four independent homozygous lines of triple mutants ( lac19 lac25 lac32 , Supplementary Fig. 15c, d ), five independent homozygous lines of double mutants ( lac25 lac32 , Supplementary Fig. 15e, f ), and single mutant of lac19 (Supplementary Fig. 15g, h ; Supplementary Data 2 ). We analyzed the phenotypes of the mutants and overexpression poplars and found the triple mutants and double mutants showed both significantly increased plant height and diameter, while lac19 showed slightly enhanced growth compare to the WT (Fig. 5a, e, f ). The two-month-old tissue cultured lac19 lac25 lac32 (Fig. 6a-c ) also showed similar phenotypes to the soil-grown poplars. However, the three laccase overexpression poplars showed decreased plant height and basal stem diameter compared with WT (Fig. 5b, g, h ). Fig. 5: lac19 lac25 lac32 poplar shows enhanced growth. a , b Growth phenotypes of lac mutants ( a ) and overexpression ( b ) poplars. Scale bar, 15 cm. ( c , d ) Phloroglucinol staining analysis of lac mutants ( c ) and overexpression ( d ) poplars. Scale bar, 40 μm. Compared with the WT, the cell walls of triple and double mutants showed lighter lignin staining and looser cell arrangement, with degrees of vessel collapse. Six samples each were analyzed with similar results. The images on the left represent CRISPR/Cas9-mediated-knockout ( c ) and 35S-mediated-overexpression ( d ), respectively. The blue asterisks represent collapsed vessels. e– h Comparisons of plant height ( e, g ) and basal stem diameter ( f, h ) for the lac mutants ( a ) and overexpression ( b ) poplars. The upper and lower whiskers represent the maximum and minimum values, respectively. The upper, lower and middle box lines represent the two quartiles and median of values in each group. All P -values are from two-tailed Student’s t -tests, and n represents 15 trees sampled respectively from each line in e, f, g, h . Source data are provided as a Source Data file. Full size image Fig. 6: The lac19 lac25 lc32 triple mutant shows enhanced saccharification efficiency. a Growth phenotypes of lac19 lac25 lc32 triple mutant. Bar, 40 mm. b , c Statistics analysis of plant height ( b ) and basal diameter ( c ) of the poplar plants ( a ). The upper and lower whiskers represent the maximum and minimum values, respectively. The upper, lower and middlebox lines represent the two quartiles and median of values in each group. All P -values are from two-tailed Student’s t -tests, and n represents 10 trees sampled respectively from each line. d Fluorescence microscopy of cell walls of WT, lac19 lac25 lac32 , lac25 lac32 , lac19 lines exposed to Tr CBM1-GFP. Tr CBM1 specifically recognizes cellulose and the probe exhibits green fluorescence. Autofluorescence (red) under UV shows lignin and the merged images highlight the negative correlation between probe binding and autofluorescence. Pf, phloem fiber; xy, xylem. Scale bars, 20 μm. e Histograms showing relative green fluorescence intensity of Tr CBM1-GFP. Values are means ± SD ( n = 3. All P -values are from two-tailed Student’s t -tests. n represents 3 trees sampled respectively from WT and the mutants). f CRM images of lac19 lac25 lac32 vessels, showing lignin deposition. Scale bars, 10 μm. Arrows indicate cell corners of WT and lac19 lac25 lac32 tested in g . g Spectra analysis of vessel cell corners in f . The grey dotted-line box represents lignin Raman spectra and is enlarged in the right panel of g . h A proposed model for the role of miR408 in regulating poplar lignification and saccharification efficiency. Monolignols are synthesized in the cytoplasm and then exported to the apoplast, oxidized and integrated into the secondary cell wall. This polymerization process is initiated by laccases, which can be down-regulated by miR408 . When LAC19, LAC25 and LAC32 were down-regulated, the polymerization of monolignols is repressed, resulting in decreased lignin content and molecular weight, leading to less polymer–polymer cross-linking of lignin and cellulose, and exposing more cellulose scaffold, with increased wall porosity and reduced wall cohesiveness, which allows increased enzyme access to biomass during saccharification in miR408_OX poplar. Source data are provided as a Source Data file. Full size image To further address laccase function in cell wall lignification, we analyzed cross-sections of basal stems with phloroglucinol staining. Compared with the WT, lac25 lac32 showed lighter lignin staining, and loose cell arrangement with a degree of vessel collapse (Fig. 5c ). The cell walls of lac19 lac25 lac32 showed more greatly decreased lignin staining, an even looser cell arrangement, and serious vessel collapse. The cell wall morphology of the single gene mutants of lac19 was not as obvious as that of the triple and double mutants (Fig. 5c ). The cell morphology of the double and triple laccase mutants was similar to that of the miR408_OX poplars. In contrast, LAC19_OX , LAC25_OX and LAC32_OX exhibited neatly arranged xylem cells, with similar morphology to WT (Fig. 5d ). Compared with the WT, the three LAC overexpression transgenic lines showed stronger staining (Fig. 5d ). Klason analysis showed lignin content of the LAC19_OX , LAC25_OX and LAC32_OX plants were increased by 19.69%, 10.67% and 14.62% respectively (Supplementary Table 2 ). To explore whether laccases are the key target for enhancing saccharification efficiency of miR408_OX poplars, cell wall accessibility of cellulose microfibrils to cellulase enzymes of the lac mutants was determined, using untreated basal stem cell walls of two-month-old tissue cultured poplars. In Tr CBM1-GFP binding experiments, the lac19 lac25 lac32 lines showed significantly increased green fluorescence signal compared with WT in both phloem fiber and xylem, the lac19 lac25 lines also showed increased green fluorescence signal, whereas lac19 poplar was similar to WT (Fig. 6d ). From the statistical analysis of fluorescence intensity, the green fluorescence signal of phloem fibers and xylem was highest in lac19 lac25 lac32 poplar (Fig. 6e ). Furthermore, lac mutants showed delayed phloem fiber development compared with WT (Fig. 6d ). In green dye-labeled cellulase enzyme binding studies, the green signal was just developing in WT (Supplementary Fig. 16a-c ) after 30 min incubation, whereas it was clearly seen in the cell walls of lac19 lac25 lac32 stems by this time (Supplementary Fig. 16d, e ). In contrast, labeling of cortical cells was much reduced in lac19 lac25 lac32 (Supplementary Fig. 16c, f ). The lac25 lac32 (Supplementary Fig. 16g-i ) lines also showed increased cell wall accessibility of cellulose microfibrils to cellulase enzymes compared with WT (Supplementary Fig. 16a-c ), whereas lac19 did not (Supplementary Fig. 16j, k ). 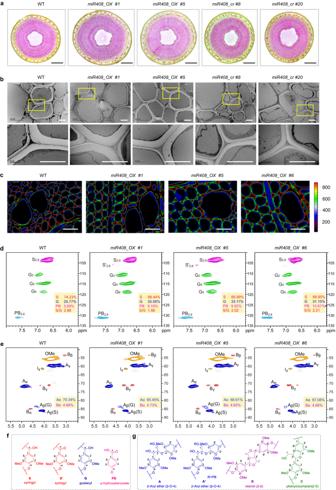Fig. 3:miR408overexpression alters lignin deposition in poplar. aCross-sections of six-month-old basal stems of WT, overexpression and knockout poplar lines. Stem cross-sections were stained with phloroglucinol-HCl (red color indicates lignin). Scale bar, 1 mm. Ten samples each were analyzed with similar results.bCell wall ultrastructure of mature xylem. Scale bar, 5 μm. Six samples each were analyzed with similar results.cCRM images of lignin in IN20 secondary xylem cell walls. The scale bar from200–800represents signal intensity from low to high. The red color represents a higher signal intensity than blue. Lignin is deposited throughout the cell wall in WT, whereas it is localized more in the corners of the cell walls ofmiR408_OXplants, indicating thatmiR408_OXplants have delayed lignification. Six samples each were analyzed with similar results.d-g2D-HQSC NMR spectra revealing aromatic regions (d,f) and lignin aliphatic side chain regions (e,g). The lignin inmiR408_OXpoplar lines had a lower relative abundance of S lignin units and a correspondingly higher abundance of G lignin units. The β-aryl ether subunits (A) were lower inmiR408_OXpoplars. The results of saccharification assays were consistent with the microscopic results (Supplementary Table 3 ). Next, we obtained CRM images (Fig. 6f ) and spectra (Fig. 6g ) to investigate changes in lignin content of vessels in lac19 lac25 lac32 and WT. The lignin distribution images were acquired by integral of the 1,545 to 1,710 cm −1 region originating from symmetrical stretching of aromatic rings. Clearly, the CRM images showed that the concentrations of lignin were highest in cell corners, and lac19 lac25 lac32 showed significantly decreased lignin deposition compared with WT (Fig. 6f, g ). Previous studies showed that over-expression miR408 can promote vegetative growth, while the impaired growth was observed in miR408 T-DNA insertion Arabidopsis mutant lines [30] . In addition, cell wall thickening was associated with the deposition of lignin and cellulose [31] , [32] . In our study, the knock-out of miR408 in poplar resulted in the enhanced cell wall lignification but the reduced cell wall thickness. Although lignin-related genes were up-regulated in the miR408 knock-out plants from the RNA-seq data, the genes encoding activators (VND7 and SND1) [33] , [34] , [35] in the transcriptional regulatory network pathway of secondary wall synthesis were down-regulated. Moreover, the expression level of LBD15 , a key TF that can down-regulate the expression of cellulose synthesis genes [36] , was increased to a large extent in miR408 knock-out poplars. The genetic evidence and gene expression analysis together suggested that miR408 may possess an additional role of regulating cell wall thickening in plants. Overexpressing miR408 in poplar contributed the enhanced plant growth associated with a significant increase in net photosynthetic rate, somewhat similar to the phenotype when overexpressing miR408 in Arabidopsis [24] . In addition, we found miR408_OX poplar showed wider cambium zone and increased xylem area (with enlarged xylem cells). We also showed that miR408 was mainly expressed in the vascular cambium and developing xylem. These results suggest a specific function for miR408 in wood formation, which is characterized by sequential differentiation of vascular cambial cells into xylem cells, cell expansion, massive deposition of secondary cell walls, programmed cell death, and ultimately, the formation of heartwood [37] , [38] . Although these anatomical features were clearly linked to miR408 overexpression or knock-out, more work is necessary to understand the coordination of the developmental and biochemical changes. It was worth noting that overexpression of miR408 in poplar, for both laboratory- and field-grown plants, results in a large increase in saccharification efficiency with no requirement for acid-pretreatment. Our study found that overexpression of Pag-miR408 can target Pag-LAC19,25 ,32, delay lignification, and modestly reduce lignin content, S/G ratio and degree of lignin polymerization. The lac triple mutants showed similar phenotypes in the vascular cell morphology, cell wall accessibility, and saccharification with miR408 _ OX poplars. Laccases are considered to function in the polymerization of lignin monomers, potentially at the stage of polymer initiation, and subsequently in concert with peroxidases [39] . Given that reduced degree of lignin polymerization is associated with improved lignin extractability and reduced biomass recalcitrance [40] , we speculate that the changes in lignin distribution and composition observed in the present miR408_OX plants result largely from the post-transcriptional regulation of three target LACCASES . Both decreased lignin polymer size and delayed lignification in miR408_OX indicated a mechanistic basis for the improved saccharification efficiency, which is enhanced by the altered ultrastructure of the vascular tissues, brought about by delayed secondary cell wall deposition during development. As shown by the increased accessibility of vascular tissues to C. thermocellum CBMs and fungal cellulase, we can conclude that the high saccharification efficiency of miR408_OX plants was largely linked to the more open cell walls for (downstream) deconstruction process. Carbohydrates found in lignocellulose (cellulose and hemicellulose) are an abundant and unused source of raw material for producing commodity chemicals such as ethanol. Depending on the gene target and extent of down-regulation, targeting monolignol biosynthetic genes can improve saccharification efficiency with or without negative impacts on biomass [6] , [10] , [41] , [42] , [43] , but seldom if ever with positive impacts. Lignification and growth are opposing processes competing for cellular resources. Here we demonstrate that it is possible to engineer directionally opposite changes in these two processes with a single transgene. In the model in Fig. 6h , we suggest that the decreased recalcitrance phenotypes and enhanced growth of the miR408_OX biomass result from repressed polymerization of monolignols, leading to less polymer–polymer cross-linking of lignin, increased wall porosity and reduced wall cohesiveness, which together increase enzyme access to biomass during saccharification. On the other hand, the looser microfibril structure may be easier to expand when the cell is growing under turgor pressure. In conclusion, down-regulating multiple laccases through targeting of specific miRNAs may be a promising way to enhance biomass saccharification through reducing lignin polymerization. These findings, which are translatable to the field, can facilitate generation of improved tree feedstocks coupling enhanced saccharification efficiency with high total biomass, providing a promising and effective approach to the production of lignocellulosic bioenergy. Plant materials and growth conditions The hybrid poplar ‘84 K’ ( Populus alba × P. glandulosa ) was used for genetic transformation. After transgenic plants were generated, screened, and verified, they were grown in a phytotron for 3, 6 and 12 months with a photoperiod of 16 h/8 h (light/dark) at 22 °C before detailed characterization. The miR408_OX and WT poplars were grown in a field plot on Beijing Forestry University field garden (40.01° N,116.35° E). After one-year growth, the plant height and basal stem diameter were measured and poplars were harvested for saccharification efficiency analysis. Plasmid construction and plant transformation Genomic sequences containing Pag- pre -miR408 on chromosome 2 were amplified via PCR from genomic DNA isolated from 84 K. The fidelity of the Pag- pre -miR408 , the CDS of LAC19 , LAC25 and LAC32 amplification was confirmed by sequencing and it was inserted into pCAMBIA2300 using Bam H I and Kpn I (Clontech) driven by the CaMV35S promoter. The 2000 bp Pag-miR408 promoter region was amplified by PCR using the primers Pag - miR408 pro-F and Pag - miR408 pro-R to create Pag-miR408 pro::GUS , which was inserted into pBI101 using Xma I and Sal I (Clontech), and confirmed by sequencing. To generate CRISPR-Cas9 miR408 knock-out poplars ( miR408_cr ), four sgRNAs were designed, two upstream and two downstream, using CCTop-CRISPR/Cas9 target online predictor ( https://cctop.cos.uni-heidelberg.de:8043/ ). The miR408 -knockout vector harboring a GUS marker gene for easily identification of positive poplars. The DNA fragments encoding the selected sgRNAs1, 2, 3 and 4 were as follows: 5’-GAGAAGGCTGAGGCTTTGAGAGG-3’, 5’-GGAAGCACAATGAAAGGTGAAGG-3’, 5’-CCTCCCTTCTTTTGTTTCCATTA-3’, 5’-GAGCGAAATATAACAGCAGCAGG-3’. To knock out LAC19 , LAC25 and LAC32 ( LACs _ cr ) at the same time, four sgRNAs1, 2, 3, 4 were designed: 5’-CGTCTCTCTTTGTTCTTCTTGGG-3’, 5’- GTCTTGCACAGCCTCTTCACTGG −3’, 5’- CTGCTTCAGAGAAATGAGCTTGG −3’, 5’- GTTCTGCACAGCCTCTTCACTGG −3’. The sgRNA2 can knock out LAC19 and LAC25 at the same time. The miR408_OX , miR408_cr , LACs_OX and LACs _ cr and pmiR408::GUS fusion vectors were introduced into Agrobacterium tumefaciens GV3101 for transformation. To provide a positive control, we generated poplar lines with lack of expression of the cinnamoyl CoA reductase CCR2 gene through RNAi. To generate the PtCCR2 -RNAi line, the amplified fragment of Pag-CCR2 was cloned into PK7GWIWG2(II)RR vector by Gateway LR reaction. The two-month-old CCR2 -RNAi tissue cultured line showed nearly 40% reduced plant height and 50% reduced stem diameter. All the primers shown in Supplementary Data 3 were synthesized by BGI. White Co., Ltd. All the constructs were transformed into ‘84 K’ by the A. tumefaciens -mediated leaf disc method according to a previous protocol [44] . For the sequence of all the mutants, the genome sequence including the targets were amplified and inserted into pGM-T. Primers are shown in Supplementary Data 3 . RNA isolation and quantitative real-time PCR To determine the expression pattern of miR408 , young leaves (first to third from the top), mature leaves (fifteenth from the top), young stems (first to third from the top), and tissues of the phloem, vascular cambium, developing secondary xylem and mature xylem from internodes 11 − 14 of six-month-old vigorously growing ‘84 K’ poplars were harvested and stored in liquid nitrogen until use. Total RNA, including small RNAs, was isolated using an RNA isolation kit (TIANGEN, DP501). Reverse transcription was performed using a First-Strand cDNA Synthesis Kit (TIANGEN, KR211). Specific primers were designed for analysis of Pag - miR408 transcript levels (Supplementary Data 3 ). 5 S rRNA was used as the endogenous control to normalize the relative expression levels of miR408 . qRT-PCR was performed using SYBR Green Mix (TIANGEN, FP401). For miRNA targets, the forward and reverse primers were designed upstream and downstream of the cleavage site. 18 S RNA from P. trichocarpa was used as an endogenous reference. In each reaction, 0.3 mM primer and 10 ng cDNA were used. For each of three biological replicates, PCR was performed in triplicate. The initial denaturing time was 30 s, followed by 40 cycles of 95 °C for 15 s, 60 °C for 15 s, and 72 °C for 15 s, with a final extension at 72 °C for 10 min. A melting curve was performed after the PCR cycles. All primer sequences are shown in Supplementary Data 3 . RNA-seq analysis RNA-seq analysis was performed with total RNA isolated from differentiating stem xylem of six-month-old poplars. Stems from three different poplar plants were pooled as one biological replicate. The transcriptome data were analyzed according to a previously described method [45] . Briefly, RNA-Seq data were generated with an Illumina HiSeq 2000 instrument at Novogene Ltd. (Beijing, China). The cleaned reads were mapped to the P . trichocarpa genome v3.1 ( https://phytozome-next.jgi.doe.gov/info/Ptrichocarpa_v3_1 ) using the Hisat2 algorithm. The gene expression levels were calculated using Fragments Per Kilobase of exon model per Million mapped fragments (FPKM) method. Cytoscape v3.7.1 software was used for miRNAs - LACs network visualization ( https://cytoscape.org/ ). The heatmaps were generated by using the GraphPad Prism v8.3 software ( https://www.graphpad.com ). Determination of saccharification efficiency Cell wall residues (CWR) generated for lignin analysis were also used to analyze the amount of total sugar. Cell wall residue refers to the cell wall material extracted by methanol and chloroform after grinding through a 40-mesh sieve. The specific extraction process is as follows: cell wall residues were generated by extracting plant tissue with methanol (three times at 37 °C for 1.5 h) and chloroform: methanol (2:1) (three times at 37 °C for 1.5 h). The samples were then washed three times with water at 37 °C for 1.5 h and lyophilized for 48 h [41] . Enzymatic saccharification of stem samples was carried out for one-year-old miR408_OX grown in the greenhouse and ten-month-old miR408_OX poplars grown in the field. For total sugar and sugar component assay, 100 ± 0.2 mg CWR was weighed into a 5 mL glass vial, 1.5 mL 72% (w/w) H 2 SO 4 added, and the mixture incubated in a water bath at 30 °C for 1 h, shaking every 10 min. Samples were transferred into 50 mL glass bottles with 42.0 mL MilliQ H 2 O, and autoclaved at 121 °C for 1 h. Materials were transferred into new 50 mL tubes, 5-10 mL Milli Q H 2 O was added, and the tubes centrifuged at 2,600× g for 30 min. The supernatants were transferred into new 50 mL tubes for sugar assay. For measuring enzyme-released sugar and sugar components without acid pretreatment, 100 ± 0.2 mg CWRs were weighed into 15 mL tubes, 10 mL Enzyme Digestion Solution added, and the tubes placed in an angled shaker and shaken at 100 rpm for 72 h at 50 °C. The tubes were centrifuged and the supernatants used for assay of released sugars [10] . The amount of fermentable sugars was analyzed using the phenol-sulfuric acid assay method [46] . Saccharification efficiency was determined as the ratio of sugars released by enzymatic hydrolysis for 72 h to the amounts of sugars present in the cell wall material before enzymatic hydrolysis. Determination of lignin content Debarked increment cores from one-year-old miR408_OX grown in the greenhouse were dried at 40 o C. After drying, the wood chips were ground in a Wiley mill with a 40-mesh screen. The resulting wood meals (40–60 mesh) were used for determination of AcBr lignin content [47] . 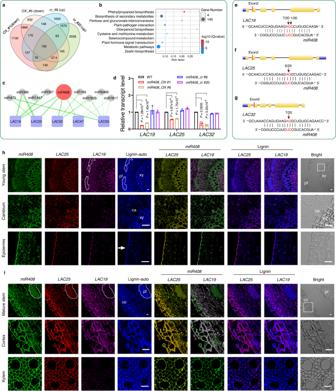Fig. 4:miR408targetsLAC19, LAC25andLAC32. aVenn diagram comparison from RNA-Seq data analysis ofmiR408_OXandmiR408_crpoplars.bKEGG pathway enrichment of DEGs that are down-regulated inmiR408_OXpoplars.cAn interaction network of five predicatedLACs(LAC19,LAC25,LAC32,LAC47andLAC55) with miR408 and other miRNAs. The thickness of the green line represents the strength of the interaction.dqRT-PCR showing the relative transcript levels ofLAC19,LAC25andLAC32with high score using psRNAtarget in WT andmiR408_OXand knockout plants. Values are means ± SD (AllP-values are from two-tailed Student’st-tests.,nrepresents 3 trees sampled respectively frommiR408_OX#1,miR408_OX#6,miR408_cr#8 andmiR408_cr#20).e–g5’RACE assays showed the cleavage site of theLAC19(e),LAC25(f) andLAC32(g). The red lines in exon 2 show the target sites, and the black arrows show the detailed miR408-guided cleavage positions.h,iLocalization ofLACsandPag-miR408using FISH method. Specific probes were designed to labelmiR408,LAC19andLAC25as green, pink and red, respectively. Lignin autofluorescence is displayed in blue. The merged images showed spatial correspondence betweenmiR408andLAC19andLAC25. In young stem (h),miR408was expressed in all the tissues, whileLAC25was highly expressed in xylem and epidermal cells, and slightly expressed in phloem cells;LAC19was only expressed in the epidermis and parenchyma cells. In mature stem (i),miR408was expressed in all the tissues, whileLAC25was highly expressed in xylem, phloem fiber and cortical cells;LAC19was expressed in cortical and parenchyma cells, but not in phloem fiber or xylem cells. Scale bar, 20 μm. Three samples each were analyzed with similar results. The dashed box represents phloem fibers. Arrows indicate the epidermis. Boxes in h and i represent the enlarged area of cambium and cortex, respectively. Source data are provided as a Source Data file. Neutral sugars in the acid-soluble fraction were derivatized to alditol acetates for quantitation by gas chromatography using a flame ionization detector (GC-FID; Agilent 7890 A) [48] . The AcBr method was used to quantify lignin content [49] . Determination of structural carbohydrates and lignin in biomass One-year-old natural debarked dried miR408_OX poplar stems grown in the greenhouse were collected. The chemical compositions (cellulosic and hemicellulosic monosaccharides and lignin) of raw material and pretreated substrates were analyzed by the standard procedure of the National Renewable Energy Laboratory (NREL) [50] . Briefly, ground (40-60 mesh) stem material (0.3 g) was placed in a tared pressure tube, 3 mL of 72% H 2 SO 4 (w/w) added, and the pressure tube placed in a water bath at 30 °C and incubated for I h. The acid was diluted to a 4% concentration by adding 84 mL deionized water using an automatic burette prior to further analysis. For carbohydrate determination, sugar recovery standards (SRS) were made by weighing out 0.1 mg of each sugar, adding 10 mL deionized water and 348 µL of 72% sulfuric acid, and transferring to a pressure tube and capping tightly. For the lignin determination, acid soluble lignin and acid insoluble lignin were determined separately [50] . Characterization of growth phenotypes For the miR408_OX and miR408_cr poplars, the growth phenotype was observed and photographed after six months of growth in the phytotron. The LACCASE overexpression and knockout poplars were photographed after three months. To investigate the anatomical structures of stems, basal stems were fixed with 2.5% (w/v) glutaraldehyde in 0.1 M cacodylate buffer (pH 7.2) for 24 h at 4 °C. The samples were then rinsed in 0.1 M cacodylate buffer, dehydrated in a graded ethanol and acetone series, infiltrated, and embedded in Spurr resin (Electron Microscopy Sciences). The resin blocks were polymerized for 24 h at 70 °C. A microtome (Leica-RM2265, Germany) was used to produce 1µm-thick sections. The sections were stained with 1% (w/v) toluidine blue and imaged using a digital camera equipped with a Leica Aperio VERSA digital pathology scanner (Leica, Germany). To analyze cell wall ultrastructure, mature xylem samples of basal stems were fixed with 2.5% (w/v) glutaraldehyde in 0.1 M cacodylate buffer (pH 7.2) for 24 h at 4 °C, rinsed in 0.1 M cacodylate buffer, and samples were fixed with 1% (w/v) osmic acid for 12 h at 4 °C. After the same embedding process, 40-nm slices were cut using an ultramicrotome and were visualized directly by transmission electron microscopy (TEM). Image-Pro Plus analysis Image-Pro Plus 6.0 (Media Cybernetics) software was used to quantify cell wall thickness, secondary xylem width, cell number and cell area [51] . GUS staining and analysis Stem sections were hand-cut and then incubated in 90 % acetone (v/v) for 10 min on ice then in GUS staining solution (100 mM sodium phosphate (pH 7.0), 10 mM EDTA, 0.5 mM ferricyanide, 0.5 mM ferrocyanide, 0.1% Triton X-100, 20 % (v/v) methanol, and 2 mM X-GLUC at 37 °C for 3 h. Following staining, sections were cleared in 95% ethanol, preserved in 75% ethanol and then photographed under the microscope (Leica DM2500, Germany). Wiesner staining Cross-sections of miR408_OX poplars were cut from stems collected after 6 months of growth to examine the increase in stem diameter using a sliding microtome (Leica SM2010 R, Germany). Stems were also collected at 3 months for tracking the development of lignification using hand-sectioning for the very young internodes and the sliding microtome for older internodes. Phloroglucinol (0.3 g, MACKLIN) was dissolved in 10 mL absolute ethanol to prepare a 3% phloroglucinol solution [52] . Fresh stem sections were placed on a slide, and 50 μL phloroglucinol solution dropped onto the section, followed by 50 μL concentrated hydrochloric acid. A cover slip was added, color development observed, and the staining photographed under the microscope (Leica DM2500, Germany). Phylogenetic analysis The amino acid sequences of 17 laccases in Arabidopsis were downloaded from the Arabidopsis information resource ( https://www.arabidopsis.org/ ). The amino acid sequences of 56 laccases in poplar were blasted from P. trichocarpa v3.1 ( https://phytozome-next.jgi.doe.gov/info/Ptrichocarpa_v3_1 ). The amino acid sequences of full-length laccases were aligned and analyzed with Clustal X 2.1 software. OrthoFinder v2.3.1 and MEGA-X 7 software were used for phylogenetic analysis [53] , with the neighbor-joining algorithm and bootstrap method of 1,000 replications. The aligned amino acid sequences used for phylogenetic analysis in Supplementary Fig. 13 are presented in Supplementary Data 4 . Assay of laccase protein level s Equal samples of fresh poplar stems of not less than 50 mg were accurately weighed. A corresponding volume (10% tissue homogenate ratio, w/v) of extraction buffer (10 mM PBS, pH 7.2–7.4) was then added and the stem samples were thoroughly homogenized. The homogenate was centrifuged twice at 4 °C for 10 min each, at 13,000× g and the sediment discarded. The supernatant was centrifuged at 4 °C for 15 min at 13,000× g . The supernatant represents the isolated stem protein extract. A double antibody sandwich ELISA assay was used to detect laccase protein level according to the manufacturer’s instructions (MEIMIAN). Raman analysis Raman spectra and Raman mapping were acquired/performed with a Via-Reflex 532/XYZ confocal Raman system (Renishaw, Great Britain). Fresh samples of 3-month-old WT and miR408_OX plants were cut into approximately 10-μm-thick sections using a sliding microtome (Leica SM2010 R). The cross-sections were focused with 532 nm laser beams and the 50× objective was used for spectroscopic analysis. The laser power on the sample was approximately 5 mW. The Raman light was detected by an air-cooled spectroscopic CCD, and the output wavelengths of the optical parametric oscillators were selected at the 1,600 cm −1 lignin aromatic ring vibration. An integration time of 1 s and a mapping step of 0.5 mm for a 10 × 10 mm region were chosen and each pixel corresponded to one scan. SRS microscopy Cross-sections of 50 μm thickness were cut at internodes IN5, IN9, IN15 and IN20 from miR408_OX poplars, using a razor blade. The SRS imaging microscope using a mode-locked Nd: YVO4 laser (High Q Laser) was used to generate a 7 ps, 76 MHz pulse train of both 1,064 nm (1 W average power) and 532 nm (5 W average power) laser beams. The 1,064 nm output was used as the Stokes light. The 532 nm beam was 50/50 split to pump two optical parametric oscillators (Levante Emerald, A · P · E Angewandte Physik und Elektronik GmbH). The output wavelength of the optical parametric oscillators was at 909 nm to use as pump beam to induce the Stimulated Raman signal for the 1,600 cm −1 lignin aromatic ring vibration. All pump and Stokes beams were directed into an Olympus laser scanning microscope scanning unit (BX62WI/FV300; Olympus) and focused by a high numerical aperture water-immersion objective (UPLSApo 60×1.20 NA W; Olympus). The light transmitted through the sample was collected by an oil-immersion condenser (1.45 NAO; Nikon). The stimulated Raman loss signals were detected by silicon PIN photodiodes (FDS1010; Thorlabs) and a lock-in amplifier (SR844; Stanford Research Systems) [54] . For each type of plant sample, at least three images were selected for intensity analysis. About 50 cells were selected and the average intensity for selected cells was calculated. In vitro transactivation assays For the vector construction, Pag-miR408 was driven by a constitutive 35 S promoter, no promoter (Nonpro) driving luciferase (LUC) was the negative control, and proActin2 driving LUC was the positive control. At the predicted binding site of target LACs and miR408 , 5 nucleotides were mutated to remove the miR408 recognition site, while at the same time guaranteeing that the amino acid sequences were unchanged. The mutated CDSs of LAC19 , LAC25 and LAC32 were named ΔLAC19 , ΔLAC25 , and ΔLAC32 . The complete CDSs of LAC19 , LAC25 and LAC32 , and of ΔLAC19 , ΔLAC25 , and ΔLAC32 were fused into pGreenII 0800 + pActin2 vector. A. tumefaciens GV3101 strains harboring the different constructs were incubated in LB liquid medium containing 50 mg/L rifampicin and 50 mg/L kanamycin for 24 h to reach OD 600 = 1.0. The bacteria were spun down at 2,600 × g for 5 min and the pellets were resuspended in infiltration buffer (10 mM MgCl 2 , 10 mM MES pH 5.6, and 100 µM acetosyringone) with a final concentration of OD 600 = 0.5. The strain suspensions were kept at room temperature for 2 h before infiltration. 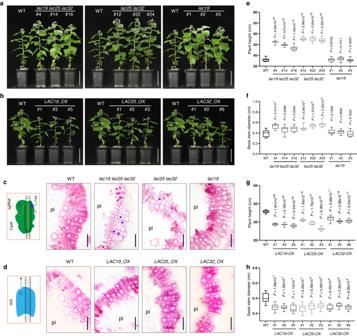Fig. 5:lac19 lac25 lac32poplar shows enhanced growth. a,bGrowth phenotypes oflacmutants (a) and overexpression (b) poplars. Scale bar, 15 cm. (c,d) Phloroglucinol staining analysis oflacmutants (c) and overexpression (d) poplars. Scale bar, 40 μm. Compared with the WT, the cell walls of triple and double mutants showed lighter lignin staining and looser cell arrangement, with degrees of vessel collapse. Six samples each were analyzed with similar results. The images on the left represent CRISPR/Cas9-mediated-knockout (c) and 35S-mediated-overexpression (d), respectively. The blue asterisks represent collapsed vessels.e–hComparisons of plant height (e,g) and basal stem diameter (f,h) for thelacmutants (a) and overexpression (b) poplars. The upper and lower whiskers represent the maximum and minimum values, respectively. The upper, lower and middle box lines represent the two quartiles and median of values in each group. AllP-values are from two-tailed Student’st-tests, andnrepresents 15 trees sampled respectively from each line ine,f,g,h. Source data are provided as a Source Data file. 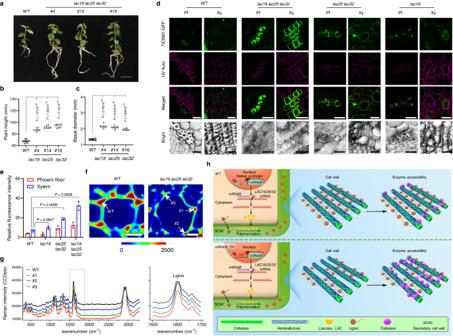Fig. 6: Thelac19 lac25 lc32triple mutant shows enhanced saccharification efficiency. aGrowth phenotypes oflac19 lac25 lc32triple mutant. Bar, 40 mm.b,cStatistics analysis of plant height (b) and basal diameter (c) of the poplar plants (a). The upper and lower whiskers represent the maximum and minimum values, respectively. The upper, lower and middlebox lines represent the two quartiles and median of values in each group. AllP-values are from two-tailed Student’st-tests, and n represents 10 trees sampled respectively from each line.dFluorescence microscopy of cell walls of WT,lac19 lac25 lac32,lac25 lac32,lac19lines exposed toTrCBM1-GFP.TrCBM1 specifically recognizes cellulose and the probe exhibits green fluorescence. Autofluorescence (red) under UV shows lignin and the merged images highlight the negative correlation between probe binding and autofluorescence. Pf, phloem fiber; xy, xylem. Scale bars, 20 μm.eHistograms showing relative green fluorescence intensity ofTrCBM1-GFP. Values are means ± SD (n= 3. AllP-values are from two-tailed Student’st-tests.nrepresents 3 trees sampled respectively from WT and the mutants).fCRM images oflac19 lac25 lac32vessels, showing lignin deposition. Scale bars, 10 μm. Arrows indicate cell corners of WT andlac19 lac25 lac32tested ing.gSpectra analysis of vessel cell corners inf. The grey dotted-line box represents lignin Raman spectra and is enlarged in the right panel ofg.hA proposed model for the role ofmiR408in regulating poplar lignification and saccharification efficiency. Monolignols are synthesized in the cytoplasm and then exported to the apoplast, oxidized and integrated into the secondary cell wall. This polymerization process is initiated by laccases, which can be down-regulated bymiR408. WhenLAC19, LAC25 and LAC32were down-regulated, the polymerization of monolignols is repressed, resulting in decreased lignin content and molecular weight, leading to less polymer–polymer cross-linking of lignin and cellulose, and exposing more cellulose scaffold, with increased wall porosity and reduced wall cohesiveness, which allows increased enzyme access to biomass during saccharification inmiR408_OXpoplar. Source data are provided as a Source Data file. For co-infiltration, equal volumes of two different strains carrying miR408_OX and LAC-LUC constructs were mixed prior to infiltration. The bacteria were infiltrated into N. benthamiana leaves using a 1 mL disposable syringe. After 72 h, the infiltrated leaves were sprayed with luciferin, and the fluorescence was detected by CCD camera (Vilber NEWTON7.0). Binding of CBM-GFP and cellulase to stem cross-sections Basal stems of two-month-old tissue cultured poplars and one-year-old natural dried poplars of miR408_OX poplars were examined. A single-blade razor was used to prepare hand-cut transverse sections. All stem sections were examined under a bright field light microscope to select samples with relatively uniform cutting and a thickness of approximately 25-30 µm. The Ct CBM3-GFP contains an N-terminal 6xHis tag, a CBM, a short linker sequence (VPVEK) and a GFP. Tr CBM1 is a family 1 CBM, also containing a sequence encoding an N-terminal 6xHis tag. The C-terminal GFP tagged Ct CBM3 sequence was synthesized (RuiBiotech) with genetic code optimization for expression in Escherichia coli . The synthesized DNA fragment was amplified by PCR using the forward primer Ct CBM3-F: 5′-GTTTAACTTTAAGAAGGAGATATACATATGACCATGATTACGCCAAGCTTGCATGCC-3′, and the reverse primer Ct CBM3-R: 5′-GAAAAGTTCTTCTCCTTTACTCATTTTTTCTACCGGTACCAGGCACTGGGAGTAGTACG-3′, Tr CBM1-F: 5′- GTTTAACTTTAAGAAGGAGATATACATATGACCATGATTACGCCAAGCTTGCATGCCC-3′, Tr CBM1-R: 5′- CTCAGTGGTGGTGGTGGTGGTGCTCGAGTTATTTGTAGAGCTCATCCATGCCATGTG-3′ and inserted into pET21a vector using the seamless cloning method. The generated Ct CBM3-GFP and Tr CBM1-GFP expression plasmids were expressed in the E. coli strain BL21 (Novagen). Fusion proteins were purified through Ni-NTA column affinity chromatography (GE Healthcare). The Ct CBM3-GFP and Tr CBM1-GFP concentration was measured by NanoDrop™ 3300 (Thermo Scientific, Wilmington, DE, USA). The working concentration of purified Ct CBM3-GFP and Tr CBM1-GFP was 0.5 mg/mL [54] , and the GFP-tagged proteins were stored in 20 mM Tris buffer (pH 8.0) at 4 o C. A commercial cellulase mixture was purchased from Yakult (Cellulase RS, Yakult, Japan). The cellulase was labeled according to the instructions supplied with the Alexa Fluor® 488 protein labeling kit (A10235, Invitrogen, Carlsbad, CA USA). For cell wall binding, 50 µL GFP-tagged Ct CBM3-GFP and Tr CBM1-GFP labeled cellulase were added to a piece of stem transverse section, incubated at room temperature for 30 min, and rinsed three times [54] . The labeled cell walls were imaged immediately by fluorescence microscopy (Leica DM2500, Germany). GFP and lignin were excited by a 488 nm laser and UV light, respectively. The fluorescence images were analyzed using Leica LAS X software. Determination of lignin molecular weight One-year-old miR408_OX grown in the greenhouse natural debarked dried poplars stems were used as the plant materials. To isolate double enzymatic lignin (DELs), ball-milled poplar wood powder (5 g) was suspended in 100 mL acetate buffer (pH 4.8) with loading of 2.5 mL of cellulase (100 FPU/mL). The reaction mixture was incubated at 50 °C on a rotary shaker (150 rpm) for 48 h. After that, the mixture was centrifuged, and the residual solid was washed extensively with acetate buffer (pH 4.8) and hot water and then freeze-dried. The dried residual solid was further subjected to the ball-milling process for 2 h and enzymatic hydrolysis as in the abovementioned procedures. After washing and freeze-drying, the DEL fractions were obtained [55] . To improve the solubility of the lignin macromolecules in tetrahydrofuran for gel permeation chromatography (GPC) analysis, the lignin was acetylated [55] . 20 mg of lignin fractions were completely dissolved in DMSO/N-methylimidazole (2:1, v/v, 0.9 mL). After continually shaking for 24 h at 25 °C in the dark, acetic anhydride (0.6 mL) was added and the mixture incubated for 2 h. Finally, the solution was dropped slowly into ice water (pH 2.0, 100 mL) to precipitate the acetylated lignin samples, and the material centrifuged and freeze-dried. The weight-average (Mw) and number-average (Mn) molecular weights of the acetylated lignin samples were determined by GPC. The GPC system (Agilent 1200, USA) was equipped with a UV detector (240 nm) and a PL-gel 10 μm Mixed-B 7.5 mm ID column, which was calibrated with monodisperse PL polystyrene standards (1390, 4830, 9970, 29150, 69650 g/mol). Four milligrams of acetylated lignin sample were dissolved in 2 mL of tetrahydrofuran (THF), and 10 μL of this solution was injected into a vial for testing. The column was operated at ambient temperature and eluted with THF at a flow rate of 1 mL min −1 . NMR sample preparation and NMR experiments 2D-HSQC NMR spectroscopy was performed on isolated (double enzymatic) lignin from stems of mature one-year-old miR408_OX grown in the greenhouse [56] . Fresh samples of 6-month-old stems of WT and miR408_OX plants were dried at 60 °C for 24 h and then stored in plastic bags before use. 5 g of each wood sample was smashed to obtain 20-40 mesh wood meal samples and was then milled in a planetary ball mill (Fritsch GmbH, Idar-Oberstein, Germany) at a fixed frequency of 500 rpm for 5 h. To prepare high-yield of double enzymatic lignin (DEL) from WT and miR408_OX poplar woods for NMR analysis, the ball-milled samples were subjected to double ball-milling and enzymatic hydrolysis according to the method as described in the first paragraph of “Determination of lignin molecular weight”. About 20 mg of DEL was dissolved in 0.5 mL of DMSO- d 6 (99.8% D). For quantitative 2D-HSQC spectra, the Bruker standard pulse program hsqcetgpsi2 was used. The spectral widths were 5000 Hz and 20000 Hz for the 1 H- and 13 C-dimensions, respectively. The number of collected complex points was 1024 for 1 H-dimension with a recycle delay of 1.5 s. The number of transients was 64-and 256-time increments were always recorded in the 13 C-dimension. The 1 J CH used was 145 Hz. Prior to Fourier transformation, the data matrixes were zero filled up to 1024 points in the 13 C-dimension. Data processing was performed using standard Bruker Topspin-NMR software. The aromatic region of the S lignin and G lignin subunits was detected by the signals around 103.8/6.67 (S2/6), 106.4/7.38 (S'2/6), 110.5/6.94 (G2), 114.8/6.88 (G5) and 118.6/6.81 (G6) ppm, with the presence of their respective diagnostic correlation signals. A quantitative analysis of the intensities of the HSQC cross-signal was performed according to the following formula: 
    I(C_9) units =  0.5I(S_2,6)+I(G_2)
 (1) where I(S 2,6) is the integration of S 2,6 , including S and S’, I(G 2 ) is the integral value of G 2 , and I(C 9 ) represents the integral value of the aromatic ring. According to the internal standard (I(C 9 )), the amount of I( X )% could be obtained by the following formula: 
    I(X)% = I(X)/I(C_9)× 100%
 (2) where I( X ) is the integral value of α-position of A (β- O −4), B (β-β), and C (β−5), respectively. The integration was performed in the same contour level. In the aromatic region, C 2,6 -H 2,6 correlations from S units and C 2 -H 2 correlation from G units were used to estimate the S/G ratio of lignin by the following formula [56] : 
    S/G =  0.5I(S_2/6)/I(G_2)
 (3) Reporting summary Further information on research design is available in the Nature Portfolio Reporting Summary linked to this article.